Warm/cool-tone switchable thermochromic material for smart windows by orthogonally integrating properties of pillar[6]arene and ferrocene 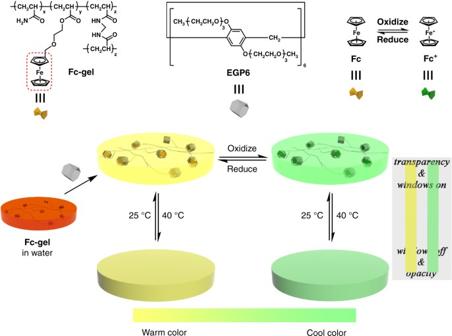Fig. 1 Chemical structures and schematic illustration of the warm/cool tone switchable thermochromic material for smart windows. Preparation ofFc-gel∙EGP6hydrogel and the schematic illustration of warm/cool tone switchable thermochromic material based on the orthogonal integration strategy of the unique properties of pillar[6]arene and ferrocene Functional materials play a vital role in the fabrication of smart windows, which can provide a more comfortable indoor environment for humans to enjoy a better lifestyle. Traditional materials for smart windows tend to possess only a single functionality with the purpose of regulating the input of solar energy. However, different color tones also have great influences on human emotions. Herein, a strategy for orthogonal integration of different properties is proposed, namely the thermo-responsiveness of ethylene glycol-modified pillar[6]arene ( EGP6 ) and the redox-induced reversible color switching of ferrocene/ferrocenium groups are orthogonally integrated into one system. This gives rise to a material with cooperative and non-interfering dual functions, featuring both thermochromism and warm/cool tone-switchability. Consequently, the obtained bifunctional material for fabricating smart windows can not only regulate the input of solar energy but also can provide a more comfortable color tone to improve the feelings and emotions of people in indoor environments. Smart windows have great potential as a way of improving building energy efficiency and indoor comfort, by reversibly modulating the amount of visible light and solar radiation entering into the buildings [1] , [2] , [3] , [4] , [5] . To achieve switchable optical performance of such smart windows, avoiding unnecessary energy consumption and unsatisfactory indoor environment, a large amount of prior research has been performed, which mostly focused on controlling the transmittance of windows by external stimuli, including electricity (electrochromism) [6] , [7] , [8] , [9] , [10] , light (photochromism) [11] , [12] , [13] , heat (thermochromism) [14] , [15] , [16] , and gas (gasochromism) [17] . Amongst these, thermochromic smart windows have attracted specific attention because they can automatically adjust the window transparency through weather-responsive control without extra energy input. This results in a reversible regulation of the solar transmittance (mainly in the near-infrared region), automatically adjusting the amount of solar heat entering into the buildings [18] , [19] , [20] . So far, vanadium dioxide (VO 2 ) is one of the most widely used inorganic materials for the fabrication of thermochromic smart windows, but the application of VO 2 -based smart windows is limited by many shortcomings, such as a high transition temperature (68 °C), low light transmittance, and unattractive blackness [21] , [22] , [23] . Meanwhile, to the best of our knowledge, few studies have achieved the construction of smart windows based on organic materials, and most of the known systems are limited to a regulation of solar energy input, thus only possessing a single functionality [24] , [25] , [26] , [27] , [28] , [29] , [30] . However, taking into account emotional and psychological effects, not only the amount of light input, but also the color of the light has a tremendous importance. In color science, color can be categorized into warm color, cool color, and neutral color [31] , [32] . Warm-tone colors, such as red, orange, and yellow makes people feel warm, lively, and excited, while cool-tone colors including green, blue, and purple gives us a feeling of coolness, serenity, and calmness. Smart windows that are capable of providing warm colors in winter and cool colors in summer will not only make our homes much more comfortable, but can also be beneficial to improve human emotions. Although, thermochromic supramolecular materials based on charge-transfer interactions with excellent color switchable property developed by Fang and Olson have attracted great interest and attention [33] , [34] , their application in the fabrication of smart windows has yet to be realized. Accordingly, developing an ideal warm/cool tone switchable thermochromic material for fabricating smart windows is an amazing and challenging endeavour, which could have an immediate positive effect on improving the quality of life for people throughout the world. Orthogonal self-assembly refers to an integration strategy of two or more types of non-covalent interactions with high specificity and selectivity [35] , [36] , [37] , [38] , [39] , [40] , [41] , [42] . Using this orthogonal strategy, various types of supramolecular complexes (such as ligand-receptor, host–guest) have been applied for the fabrication of smart and functional materials based on supramolecular polymers. However, up to now, most orthogonal self-assembly strategies rely on selective orthogonal supramolecular interactions, while the individual functional properties of the interacting entities are not fully explored. For example, pillar[n]arenes [43] , [44] , [45] , [46] , [47] , [48] , [49] , [50] , [51] , [52] , [53] , as a family of macrocyclic hosts, not only possess outstanding properties in host–guest chemistry, but can also undergo facile modification to introduce additional fascinating functionalities, such as hydrophobicity for super-hydrophobic surfaces [54] , water-solubility [55] , biofilm inhibition [47] , multi-responsiveness to CO 2 [56] , light [48] , temperature [57] , and so on. Inspired by the concept of orthogonal self-assembly, we try to orthogonally integrate the unique properties of different supramolecular substrates to achieve the fabrication of smart materials with cooperative and non-interfering functions. Herein, a dry gel with ferrocene pendants modifying on the polyacrylamide-based polymer networks ( Fc-gel ) has been successfully prepared. A well-swollen and high transparent hydrogel ( Fc-gel∙EGP6 ) is obtained when the Fc-gel is immersed in the aqueous solution of ethylene glycol chain-modified pillar[6]arene ( EGP6 ). This phenomenon is due to the formation of hydrophilic inclusion complexes between EGP6 and the ferrocene groups of Fc-gel instead of the original hydrophobic domains formed by physical cross-linking of the hydrophobic ferrocene units. Thus, water absorption capacity of the generated Fc-gel·EGP6 hydrogel is significantly improved, which results in a drastically improved swelling behaviour and an enhanced transparency of the Fc-gel·EGP6 hydrogel in comparision to the dry Fc-gel . Moreover, owing to the thermo-responsiveness of EGP6 and the reversible transformation between orange and green colors of ferrocene/ferrocenium groups under redox-response, we have orthogonally integrated the functional properties of both supramolecular building blocks based on host–guest interaction in order to design a warm/cool tone-switchable thermochromic material. This material is highly suitable for the fabrication of smart windows with dual functionality, both for regulating the input of solar energy and for improving the feelings and emotions of inhabitants for a comfortable life (Fig. 1 ). Fig. 1 Chemical structures and schematic illustration of the warm/cool tone switchable thermochromic material for smart windows. Preparation of Fc-gel∙EGP6 hydrogel and the schematic illustration of warm/cool tone switchable thermochromic material based on the orthogonal integration strategy of the unique properties of pillar[6]arene and ferrocene Full size image Preparing Fc-gel·EGP6 hydrogel by host–guest complexation Initially, the complexation between EGP6 and Fc -containing polymer networks was investigated by 1 H NMR spectroscopy. Since both the polymer networks and the hydrophobic ferrocene moiety are insoluble in water, a water-soluble linear polymer mPEG-Fc was selected as a model guest for the host–guest complexation study (Fig. 2 and Supplementary Fig. 2 ). When a mixture of EGP6 and mPEG-Fc with a 1:1 mole ratio was dissolved in D 2 O, the peaks for protons on EGP6 were shifted to low field, with the most significant downfield chemical shift observed for the aromatic protons H A (Δδ = 0.14 ppm). Meanwhile, the signal for the ferrocene-protons (H B , including one methylene unit) of mPEG-Fc showed an obvious upfield chemical shift (overlapped with the peaks of EGP6 ) due to the shielding effect of the electron-rich cavity of EGP6 . The above results reveal that the ferrocene moiety of model guest mPEG-Fc is threaded into the hydrophobic cavity of EGP6 . This was also confirmed by a 2D NOESY experiment (Supplementary Figs. 4 and 5 ), which clearly showed the NOE correlation signals between protons H A of EGP6 and part of protons H B on the ferrocene moiety of mPEG-Fc . Fig. 2 Host–guest complexation investigated by 1 H NMR spectroscopy. Partial 1 H NMR spectra (400 MHz, D 2 O, 298 K) of a 2 mM mPEG-Fc ; b 2 mM EGP6 and 2 mM mPEG-Fc ; c 2 mM EGP6 Full size image Subsequently, a Job’s plot analysis based on UV–vis spectra data showed that the complexation between EGP6 and the ferrocene moiety of mPEG-Fc had 1:1 stoichiometry (Supplementary Fig. 1 ). The corresponding binding constant of EGP6 ⊃ mPEG-Fc in water was determined to be (3.98 ± 0.10) × 10 2 M −1 by a non-linear curve-fitting method (Supplementary Fig. 3 ). In this case, hydrophobic interaction is the main driving forces for such a host–guest complexation, leading to the formation of a stable 1:1 inclusion complex between EGP6 and the ferrocene moiety. Having demonstrated the Fc-EGP6 interaction in the model substrate, we turned our attention to the Fc -substituted polymer networks for the following investigation. A disc-shaped sample consisting of cross-linked random copolymers ( Fc-gel ) was prepared by free radical copolymerization of acrylamide, a ferrocene-modified monomer, and N , N ′-methylenebis(acrylamide) (MBA) under conventional conditions (for details, see preparation of Fc-gel in Supplementary Discussion). Based on our previous work [55] , the obtained Fc-gel should display a significant swelling behavior in an aqueous solution of water-soluble pillar[6]arene. The swelling ratio will be dramatically promoted with an increasing amount of the incorporated ferrocene subunits from 0% to 10 mmol%; whereas, when the ferrocene loading was more than 10 mmol%, a decreased swelling ratio is expected induced by the dominant hydrophobic effect of the ferrocene groups. Therefore, in this study, the molar ratio of ferrocene subunits in Fc-gel was selected as 10 mmol% for sufficient host–guest complexation with EGP6 and subsequent excellent swelling behavior of Fc-gel . The samples of Fc-gel were immersed in water or EGP6 aqueous solution at 25 °C to investigate their different swelling behaviors. When immersed in EGP6 aqueous solution (15 mM), the dry Fc-gel showed dramatical swelling, and the diameter of the disc increased from 7 to 17.5 mm with an increment of 150% compared to the dried sample (Fig. 3c and Supplementary Fig. 6 ). Moreover, the obtained sufficiently swollen hydrogel exhibited a homogeneous morphology with a porous network structure, as observed from scanning electron microscopy (SEM) image (Fig. 3b ). In contrast, when the dry Fc-gel was immersed in pure water as a control experiment, the equilibrium diameter only increased by 64.3% (from 7 to 11.5 mm, Fig. 3c and Supplementary Fig. 6 ), and the obtained hydrogel exhibited a heterogeneous morphology with denser matrix and a non-uniform porous structures observed from the SEM image (Fig. 3a ). The main reason for this different swelling behavior can be attributed to the formation of hydrophilic EGP6 -ferrocene inclusion complexes, which transformed the hydrophobic ferrocene groups into hydrophilic moieties and resulted in the obviously improved water absorption capacity and drastically increased swelling property of the Fc-gel in the presence of EGP6 . Fig. 3 SEM micrographs and photographs of hydrogels. SEM micrographs of freeze-dried Fc-gel immersed in a pure water and b EGP6 aqueous solution (15 mM); Scale bars are 50 µm. c the corresponding photographs of Fc-gel under different conditions Full size image Fabricating orthogonal functional material for smart windows The response to external stimuli is a significant property of smart hydrogels. Since EGP6 shows a unique thermo-responsiveness [57] and the ferrocene moiety exhibits a reversible transformation between orange and green ferrocene/ferrocenium groups under redox-stimuli [55] , we envisaged the orthogonal integration of both of the above unique properties to design a warm/cool tone-switchable thermochromic material for fabricating smart windows. Initially, we investigated the stimuli-responsive properties of EGP6 and ferrocene in aqueous solution. When EGP6 aqueous solution was heated up to 40 °C, a white and turbid solution was obtained, which could return to a clear solution after being cooled to 25 °C (Fig. 4a, b ). Meanwhile, mPEG-Fc in its aqueous solution exhibited an orange color. Whereas, upon oxidization with ammonium persulfate, the original orange solution gradually became dark green due to the transformation of ferrocene into ferrocenium ( Fc + ), which could be reversed by subsequent reduction process, restoring the original orange color (Fig. 4c, d , for the host–guest interaction between Fc + and EGP6 , see Supplementary Figs. 8 – 10 ). Based on these observations, we tried to orthogonally integrate the above unique properties of EGP6 and ferrocene to the obtained hydrogel for further fabricating of a warm/cool tone-switchable thermochromic material for smart windows. Fig. 4 Stimuli-responsive properties of EGP6 and ferrocene in solution. Transparency of EGP6 aqueous solution (4 mM): a at 25 °C and b at 40 °C; colors of mPEG-Fc solution at c reduction state and d oxidation state, respectively Full size image For the construction of smart windows, transparency is one of the most important prerequisites to ensure indoor illumination and input of solar energy. Therefore, the prepared functional materials for smart windows should firstly be transparent. The obtained well-swollen Fc-gel·EGP6 hydrogel shows a high grade of transparency and an orange color, thus providing an excellent foundation for its potential application in constructing windows (Fig. 3c ). Investigation of the optical transparency of Fc-gel·EGP6 hydrogel by UV–vis transmission spectrum (Supplementary Fig. 7 ) showed enhanced transmittance with increasing wavelength in the visible region (380–780 nm) at 25 °C. More importantly, the hydrogel showed a high transmittance from 79.4 to 89.6% in the near infrared region (780–1100 nm). Thus, the Fc-gel·EGP6 hydrogel is ideally suited to allow an excellent input of solar energy, effectively increase the indoor temperature with windows prepared by such a functional material. Moreover, the orange warm-toned color of the material makes it a potential candidate for smart windows with the ability to make indoor people feel warm and lively. We next turned our attention to a possible thermo-responsiveness of the material. From an application point-of-view, we aspired to minimize the input of solar energy when the indoor temperature was too high to live comfortably. Especially in summer, thermo-responsive windows would represent an effective means of reducing the indoor temperature and thus decrease the electrical energy consumption of air conditioning devices. Therefore, we further evaluated the temperature-dependent transparency of Fc-gel·EGP6 hydrogel caused by the thermal-responsiveness of EGP6 . Upon increasing the environmental temperature to 40 °C, the Fc-gel∙EGP6 hydrogel rapidly became opaque within only 10 s (Fig. 5b and Supplementary Movie 1 ), and the transmittance of the hydrogel approached zero in the whole wavelength range (300–2000 nm) (Fig. 6b and Supplementary Fig. 13 ). Notably, this hydrogel material showed a good combination of higher luminous transmittance ( T lum = 64.0%) and solar modulation ability (Δ T sol = 66.9%) [58] , which was calculated according to the reference method [59] . However, in the control experiment, the Fc-gel hydrogel prepared by immersing in pure water always remained its transparent in a temperature range from 25 to 45 °C without any changes in transmittance (Figs. 5a and 6a ). This phenomenon is based on the thermal-responsiveness of EGP6 . At low temperatures, the Fc-gel·EGP6 hydrogel will be formed driven by host–guest interaction. However, upon increasing the temperatures above its cloud point temperature ( T cloud ), EGP6 will aggregate and microseparate from water inside the hydrogel due to the interaction of the hydrophobic groups of pillararene backbone [57] , and finally, resulting in the generation of an opaque Fc-gel∙EGP6 hydrogel with the ability to prevent visible light and solar radiation from passing through. When decreasing the temperature from 40 to 25 °C, the opaque Fc-gel·EGP6 hydrogel immediately returned to its original transparency because of the re-dissolution of EGP6 below its T cloud (Supplementary Movie 1 ). Meanwhile, such reversible thermo-responsive behavior was also supported by variable-temperature 1 H-NMR spectroscopy (Supplementary Fig. 11 ). More importantly, after more than 100 cycles of alternating temperature increasing/decreasing, the transmittances kept almost constant between two values measured at 1099 nm (Fig. 7a ). In addition, the Fc-gel·EGP6 hydrogel remained very good stability without any leakage of EGP6 from the hydrogel backbone even after 100 thermal cycles (Supplementary Fig. 12 ). Therefore, we can confirm that the transparency/opaqueness of the Fc-gel∙EGP6 hydrogel is reversible and highly reproducible for many alternating cycles between 25 and 40 °C. Fig. 5 Warm/cool tone-switchable and thermochromic properties of the hydrogels. Transparency of a Fc-gel immersed in pure water (sample thickness 1 mm); b Fc-gel immersed in EGP6 solution (forming Fc-gel·EGP6 hydrogel, sample thickness 2.8 mm); c oxidized Fc-gel·EGP6 hydrogel at 25 °C, 35 °C, 40 °C, and 45 °C, respectively Full size image Fig. 6 Transmittance changes under different conditions. Transmittance changes of a Fc-gel immersed in pure water; b Fc-gel∙EGP6 hydrogel; d oxidized Fc-gel∙EGP6 hydrogel at 25 and 40 °C; c Fc-gel·EGP6 hydrogel before and after oxidation Full size image Fig. 7 Reproducibility of the Fc-gel·EGP6 hydrogel in warm/cool tone-switchable and thermochromic functions. Transmittance changes of a Fc-gel·EGP6 hydrogel and b oxidized Fc-gel·EGP6 hydrogel at 1099 nm by alternately exposing to water at 25 and 40 °C. c Color changes and d transmittance changes at 1099 and 620 nm of Fc-gel·EGP6 hydrogel by alternately exposing to (NH 4 ) 2 S 2 O 8 (cool color) and N 2 H 4 ·H 2 O (warm color) aqueous solution at 25 °C Full size image With regard to the second functionality of the material, the warm/cool tone color change, we subsequently investigated its reversible redox-behaviour. When the Fc-gel∙EGP6 hydrogel was immersed in ammonium persulphate aqueous solution ((NH 4 ) 2 S 2 O 8 ), the gel gradually changed its color from orange to green within 8 min (Fig. 5c and Supplementary Movie 2 ). This is mainly due to the fact that the original color of the hydrogel was contributed by the orange ferrocene group, which is transformed into green ferrocenium moiety upon oxidation (Fig. 4c, d ). To our delight, the oxidation process had hardly any impact on the transmittance of the Fc-gel·EGP6 hydrogel and the obtained oxidized hydrogel with green color also exhibited high transparency. From the UV–vis transmission spectra (Fig. 6c ), a small absorption peak at about 620 nm could be observed, giving direct spectroscopic evidence of the ferrocenium-moiety. Meanwhile, similar as the Fc-gel·EGP6 hydrogel, the oxidized hydrogel with dark green color also had excellent thermochromism (Figs. 5c and 6d , and Supplementary Movie 3 ), and the reversible transformation between transparency and opaqueness of the oxidized hydrogel were also highly reproducible for more than 100 thermal cycles (Fig. 7b ). Interestingly, a reverse process for transforming the green hydrogel into its original orange color could be achieved by immersing the oxidized hydrogel in hydrazine hydrate (N 2 H 4 ·H 2 O) aqueous solution (Supplementary Movie 2 ), leading to the reduction of green ferrocenium into orange ferrocene groups [55] . And the regenerated orange hydrogel also maintained its high transparency and good performance of thermochromism (Fig. 7d ). Moreover, the above switchable process between orange and green colors exhibited good reversibility and high repeatability based on the oxidization/reduction of the ferrocene groups within the Fc-gel·EGP6 hydrogel (Fig. 7c ). More importantly, the oxidized green Fc-gel·EGP6 hydrogel material possesses the characteristics of cool-toned colors. Thus, this material could be used to fabricate smart windows for providing cool and calm feelings of indoor people. In addition, for the real-life applications of smart windows, a feasible and practical way for affecting the desired switching process is necessary. In this Fc-gel·EGP6 hydrogel system, thermochromic performance depends on the environmental temperature, while the color switching between warm and cool tune can be controlled by a feasible redox stimuli. According to previous work [60] , [61] , [62] , cyclic voltammetry (CV) study indicated that the pillararene–ferrocene inclusion complexes have stable oxidation and reduction peaks. 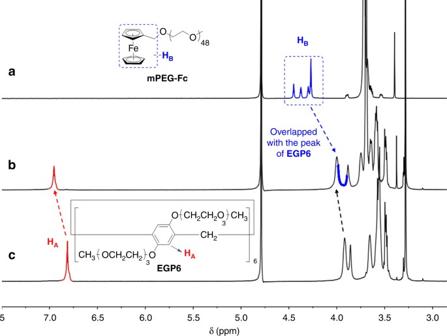Fig. 2 Host–guest complexation investigated by1H NMR spectroscopy. Partial1H NMR spectra (400 MHz, D2O, 298 K) ofa2 mMmPEG-Fc;b2 mMEGP6and 2 mMmPEG-Fc;c2 mMEGP6 Therefore, we have fabricated an electrochemical device based on the Fc-gel•EGP6 hydrogel to achieve the color switching between warm and cool tune by applying a suitable electric potential instead of using chemical oxidizing and reducing agents. As shown in Fig. 8 , after being immersed in KCl aqueous solution (0.1 M), the Fc-gel·EGP6 hydrogel was sandwiched between two pieces of ITO conductive glass to form a simple device. Upon holding the potential at +4.0 V for 6 min, the color of the material in the device could be completely transformed from orange to green due to the electrochemical oxidation of ferrocene to ferricenium cation. After further holding the potential at –4.0 V for 6 min, the Fc-gel·EGP6 hydrogel was reduced and the color of the material returned to orange. Therefore, based on the orthogonally integrated properties of EGP6 and ferrocene by host–guest interaction, a warm/cool tone-switchable Fc-gel·EGP6 hydrogel was successfully prepared, which could be used as a novel material for fabricating smart windows to improve the emotions of indoor people, meanwhile, both in warm and cool tones, the hydrogel was transparent and possessed excellent thermochromism to control the input of solar energy for a more comfortable indoor environment. Fig. 8 An electrochemical device based on Fc-gel•EGP6 hydrogel. a Schematic illustration of the electrochemical device based on Fc-gel•EGP6 hydrogel; b Photographs of the device in reduced and oxidized states, respectively Full size image 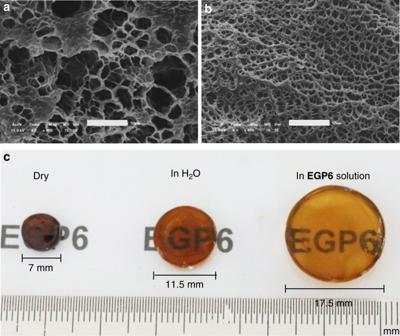Fig. 3 SEM micrographs and photographs of hydrogels. SEM micrographs of freeze-driedFc-gelimmersed inapure water andbEGP6aqueous solution (15 mM); Scale bars are 50 µm.cthe corresponding photographs ofFc-gelunder different conditions In summary, we have orthogonally integrated the unique properties of pillar[6]arene and ferrocene based on host–guest interaction to develop a warm/cool tone-switchable thermochromic material for the fabrication of smart windows. Owing to the efficient EGP6 -ferrocene complexation, a well-swollen and highly transparent Fc-gel∙EGP6 hydrogel was prepared by immersing a ferrocene-modified polyacrylamide-based polymer networks in EGP6 aqueous solution. 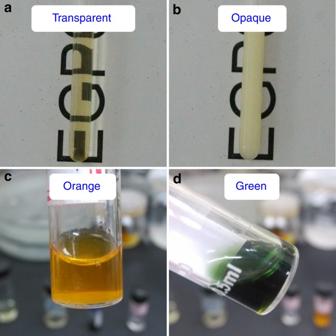Fig. 4 Stimuli-responsive properties of EGP6 and ferrocene in solution. Transparency ofEGP6aqueous solution (4 mM):aat 25 °C andbat 40 °C; colors ofmPEG-Fcsolution atcreduction state anddoxidation state, respectively Moreover, the generated Fc-gel∙EGP6 hydrogel exhibited warm/cool tone-switchable property owing to the reversible transformation between orange and green ferrocene/ferrocenium groups under redox-stimuli, which has potential applications in fabricating smart windows with specific function for improving the feelings and emotions of indoor people. More importantly, the transparent Fc-gel·EGP6 hydrogel inherited the excellent thermo-responsiveness of EGP6 in both warm and cool color to become a thermochromic material, which can regulate the input of solar energy for a more comfortable indoor environment. In this study, the unique properties of EGP6 and ferrocene were orthogonally integrated together, where both EGP6 and ferrocene perform its own duty with non-interference but mutual promotion. 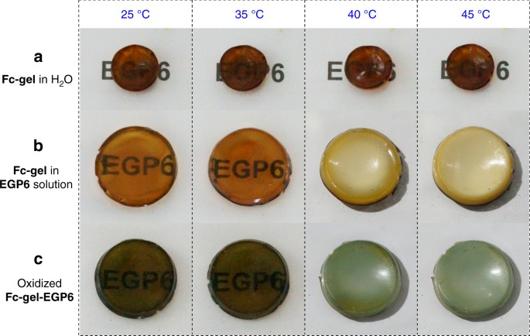Fig. 5 Warm/cool tone-switchable and thermochromic properties of the hydrogels. Transparency ofaFc-gelimmersed in pure water (sample thickness 1 mm);bFc-gelimmersed inEGP6solution (formingFc-gel·EGP6hydrogel, sample thickness 2.8 mm);coxidizedFc-gel·EGP6hydrogel at 25 °C, 35 °C, 40 °C, and 45 °C, respectively Therefore, we successfully provide the first applied example for this orthogonal integration strategy of different properties with the purpose of developing a warm/cool tone-switchable thermochromic material for fabricating smart windows, which have promising applications in the field of material science and technology. Furthermore, we believe that this orthogonal integration strategy of different properties might provide a new direction for design and development of novel functional materials. General All reagents were commercially available and used as supplied without further purification unless otherwise stated. EGP6 , mPEG-Fc ( M n = 2347 g·mol −1 ), ferrocene-modified acrylamide monomer ( FcAm ), and dry Fc-gel were synthesized according to the literatures [52] , [55] , [57] . Nuclear magnetic resonance (NMR) spectra were recorded on a Bruker Advance DMX 400 spectrophotometer or a Bruker Advance DMX 500 spectrophotometer with internal standard tetramethylsilane (TMS) and solvent signals as internal references at 25 °C. SEM was carried out on a Shimadzu SSX-550 device. 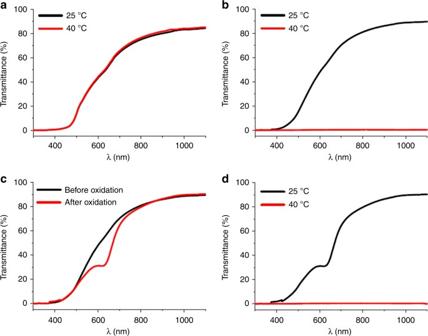Fig. 6 Transmittance changes under different conditions. Transmittance changes ofaFc-gelimmersed in pure water;bFc-gel∙EGP6hydrogel;doxidizedFc-gel∙EGP6hydrogel at 25 and 40 °C;cFc-gel·EGP6hydrogel before and after oxidation UV–vis spectra were recorded on a Shimadzu UV-1780 UV–vis Spectrophotometer. Preparation method of dry Fc-gel FcAm (220 mg, 0.70 mmol), acrylamide (448 mg, 6.30 mmol), and N , N ′-methylenebis(acrylamide) (MBA) (5.40 mg, 0.035 mmol) were dissolved in dimethyl sulfoxide (DMSO) (1.6 mL). Then azodiisobutyronitrile (AIBN) (28.8 mg, 0.175 mmol) was added to the solution and the mixture was purged with dry argon for 30 min. The resulting solution was equally divided into 10 vials (10 mm in diameter) and sealed. The polymerization was performed in an oven at 70 °C for 24 h. Then, the vials were cooled down to room temperature, disc-shaped samples were washed successively by DMSO and deionized water, and subsequently dried in oven (50 °C) under vacuum for 12 h after natural drying. Finally, disc-shaped dry Fc-gel was obtained with 7 mm in diameter and 1 mm in thickness. Synthesis and characterization Synthesis and relevant characterization details are provided in the Supplementary Information . Data availability The authors declare that the data supporting the findings of this study are available within the paper and its Supplementary Information including Supplementary Methods and Supplementary Discussion . 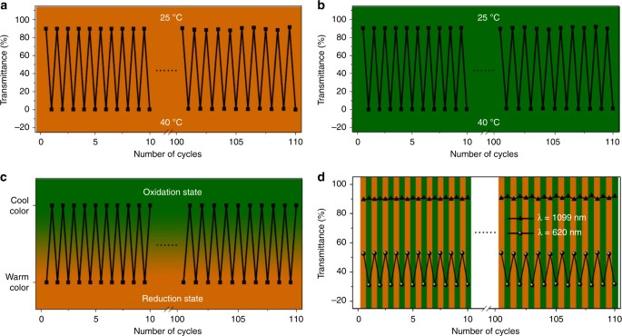Fig. 7 Reproducibility of theFc-gel·EGP6hydrogel in warm/cool tone-switchable and thermochromic functions. Transmittance changes ofaFc-gel·EGP6hydrogel andboxidizedFc-gel·EGP6hydrogel at 1099 nm by alternately exposing to water at 25 and 40 °C.cColor changes anddtransmittance changes at 1099 and 620 nm ofFc-gel·EGP6hydrogel by alternately exposing to (NH4)2S2O8(cool color) and N2H4·H2O (warm color) aqueous solution at 25 °C 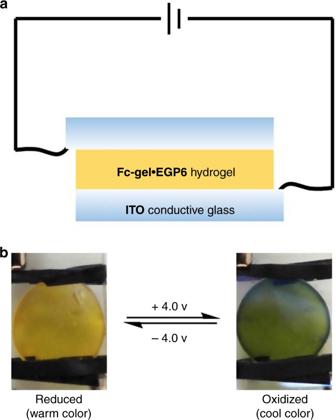Fig. 8 An electrochemical device based onFc-gel•EGP6hydrogel.aSchematic illustration of the electrochemical device based onFc-gel•EGP6hydrogel;bPhotographs of the device in reduced and oxidized states, respectively All data are available from the authors on reasonable request.